Spin transport and Hanle effect in silicon nanowires using graphene tunnel barriers Spin-based devices offer non-volatile, scalable, low power and reprogrammable functionality for emerging device technologies. Here we fabricate nanoscale spintronic devices with ferromagnetic metal/single-layer graphene tunnel barriers used to generate spin accumulation and spin currents in a silicon nanowire transport channel. We report the first observation of spin precession via the Hanle effect in both local three-terminal and non-local spin-valve geometries, providing a direct measure of spin lifetimes and confirmation of spin accumulation and pure spin transport. The use of graphene as the tunnel barrier provides a low-resistance area product contact and clean magnetic switching characteristics, because it smoothly bridges the nanowire and minimizes complicated magnetic domains that otherwise compromise the magnetic behaviour. Utilizing intrinsic two-dimensional layers such as graphene or hexagonal boron nitride as tunnel contacts on nanowires offers many advantages over conventional materials deposited by vapour deposition, enabling a path to highly scaled electronic and spintronic devices. Semiconductor nanowires (NWs) provide an avenue to further reduce the ever-shrinking dimensions of transistors [1] , and NW transistors successfully provide complex logic and sensor operation [2] , [3] , [4] . Adding electron spin as an additional state variable offers new prospects for information processing in semiconductors [5] , [6] , [7] , enabling future electronic devices beyond the current semiconductor technology roadmap [1] , [8] , [9] , [10] . Spin-based devices promise to combine the advantages of charge-based dynamic memory (speed and density) with those of magnetic storage (non-volatility, low power and radiation hardness). Silicon is an ideal host for such a spin-based technology, because its low atomic mass and crystal inversion symmetry result in very small spin–orbit interactions, promoting spin transport [5] , [6] , [11] , [12] . Silicon NWs thus provide a path to highly scaled spintronic devices [13] , [14] . Realization of spin-based Si NW devices requires efficient creation, transport and detection of spin populations and currents within the transport channel [15] . Electrical spin injection and detection depend critically on the interface resistance between the spin-injecting ferromagnetic (FM) metal contact and the semiconductor [16] . This is especially problematic with nanowires because of the exceedingly small contact area, which can be of order 100 nm 2 (refs 17 , 18 ). Oxide tunnel barriers circumvent the metal/semiconductor conductivity mismatch and enable good spin injection into planar Si structures [19] , [20] , [21] , [22] , [23] , [24] , [25] , but such contacts grown on our nanowires were found too resistive to yield reliable and consistent results. We have previously shown that single-layer graphene forms low-resistance area (RA) product tunnel barriers on bulk Si, while providing spin-injecting properties superior to those of oxide tunnel barriers [26] . Graphene’s unique properties [27] also prevent diffusion and the formation of silicides [28] . Here we fabricate nanoscale spintronic devices comprised of a Si nanowire channel with low-resistance graphene tunnel barriers for electrical spin injection and detection of pure spin currents. We use both four-terminal non-local spin-valve (NLSV) [29] , [30] and three-terminal (3T) [31] geometries to probe spin accumulation and transport. In contrast with previous work [32] , [33] , [34] , [35] , [36] , we observe Hanle spin precession in both measurements. Because spurious effects can produce spin-valve-like behaviour even in the non-local geometry [37] , the Hanle effect is widely regarded as the gold standard for spin transport [15] . Our Hanle data provide confirmation of spin accumulation and pure spin transport, enabling direct measurements of spin lifetimes and diffusion lengths in these device configurations. Graphene provides a low-resistance area product tunnel barrier contact, and minimizes complicated magnetic domains that otherwise compromise the magnetic behaviour [33] . Fabrication of nanowire spin-valve devices Si nanowires were grown using gold seeded vapour–liquid–solid techniques with a <111> growth axis (see Methods section) [38] . The wires were phosphorous doped to an electron concentration n ∼ 3 × 10 19 cm −3 . They were removed from the growth substrate by sonication and dispersed on a Si 3 N 4 /Si substrate. Appropriate nanowires ∼ 100–150 nm in diameter were chosen optically, and two outer ohmic contacts were made using electron-beam lithography. A buffered hydrofluoric acid-based solution was used to remove any thin oxide layer and hydrogen passivate the nanowires. Graphene grown by low-pressure chemical vapour deposition within Cu foil enclosures [39] was transferred onto the hydrogen-passivated nanowires using mechanical transfer techniques. The magnetic contacts, Au 300 Å/NiFe 100 Å, were defined by electron-beam lithography using PMMA resist and deposited by electron-beam evaporation to form the devices illustrated in Fig. 1a on which both 3T and NLSV measurements could be made. These magnetic contacts, labelled 2 and 3, are 1 μm and 200 nm wide, respectively, separated edge-to-edge by 200 nm. The different contact widths insure different coercive fields for the NLSV measurements. These contacts are then used as a hard mask to remove the excess graphene by a light O 2 plasma etch. Complete removal of excess graphene was confirmed when the resistance between these electrodes increased by three orders of magnitude. 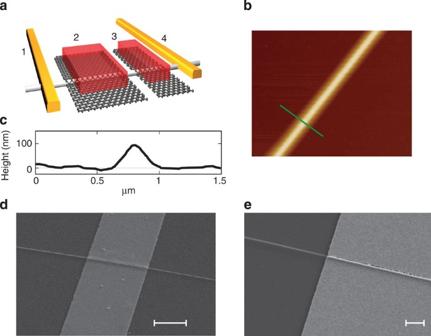Figure 1: Fabrication of graphene/nanowire structures. (a) Schematic of four-terminal nanowire device; contacts 1 and 4 are ohmic contacts applied directly to the nanowire, and contacts 2 (1 μm wide) and 3 (200 nm wide) are NiFe/graphene tunnel barriers for electrical spin injection and detection. The edge-to-edge separation of contacts 2 and 3 is 200 nm. (b) Atomic force microscopy image of graphene covered nano wire, green line is line scan shown inc, (c) line scan of graphene covered nanowire. (d) Scanning electron microscopy (SEM) image of a NiFe/graphene contact on NW. The graphene smoothly bridges the nanowire so that the NiFe film is smooth and continuous. Scale bar, 1 μm. (e) SEM image of an Au contact on an NW showing discontinuous portions of the metallization at the nanowire. Scale bar, 1 μm. Figure 1: Fabrication of graphene/nanowire structures. ( a ) Schematic of four-terminal nanowire device; contacts 1 and 4 are ohmic contacts applied directly to the nanowire, and contacts 2 (1 μm wide) and 3 (200 nm wide) are NiFe/graphene tunnel barriers for electrical spin injection and detection. The edge-to-edge separation of contacts 2 and 3 is 200 nm. ( b ) Atomic force microscopy image of graphene covered nano wire, green line is line scan shown in c , ( c ) line scan of graphene covered nanowire. ( d ) Scanning electron microscopy (SEM) image of a NiFe/graphene contact on NW. The graphene smoothly bridges the nanowire so that the NiFe film is smooth and continuous. Scale bar, 1 μm. ( e ) SEM image of an Au contact on an NW showing discontinuous portions of the metallization at the nanowire. Scale bar, 1 μm. Full size image Tunnel barrier contact characterization Figure 1b shows an atomic force microscopy image of the wire and Fig. 1c shows a corresponding line scan across the wire directly after the graphene transfer onto a 100-nm diameter Si nanowire. As reported in ref. 40 , the graphene smoothly bridges the nanowire and forms freely suspended graphene for approximately the width of the nanowire on each side, like a blanket on a clothesline. This free-hanging graphene is robust to electron-beam evaporation of NiFe, and produces a smooth and continuous NiFe film across the nanowire as is evident from the scanning electron microscopy image in Fig. 1d . The smooth bridging provided by graphene results in clean switching of the contact magnetization as discussed below, because it minimizes the formation of complicated magnetic domains that have been found to compromise the magnetic behaviour and complicate interpretation of the resulting data [33] . In contrast, the scanning electron microscopy image of the Au reference contact, Fig. 1e , shows that this metal layer without graphene underneath attempts to be highly conformal to the NW, resulting in discontinuous portions of the metallization. These contacts were initially characterized using current–voltage ( I–V) measurements. 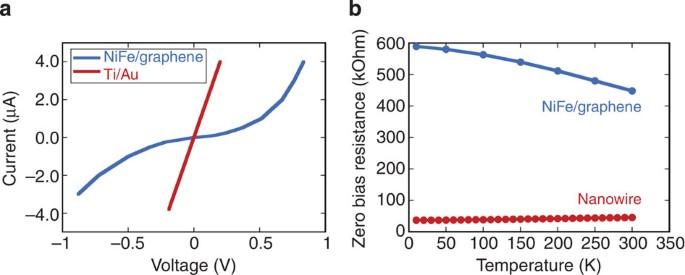Figure 2: Electrical characterization of tunnel contacts. (a)I–Vcurves of the Au/Ti/150 nm nanowire/Ti/Au contact circuit (red) and the NiFe (7.5 μm wide)/Graphene/150 nm nanowire/Ti/Au contact circuit (blue) at 10 K. (b) Temperature dependence of zero-bias resistance for the NiFe/graphene contact (weakly insulating) and Au/Ti contact (metallic). Figure 2a shows the I–V curves of the Au/Ti/nanowire reference contacts (red) and the Au/NiFe/graphene/nanowire contacts (blue). The former are linear and have a temperature dependence of the zero-bias resistance (zbr) that is metallic in character, with the zbr increasing slightly at higher temperatures as shown in Fig. 2b . In contrast, the I–V curve of the Au/NiFe/graphene/nanowire contact is non-linear, with a parabolic bias dependence of its conductance. The corresponding zbr decreases slightly with increasing temperature, and exhibits a weak temperature dependence as shown in Fig. 2b , demonstrating that this contact is a high-quality, pinhole free tunnel barrier [41] . Figure 2: Electrical characterization of tunnel contacts. ( a ) I–V curves of the Au/Ti/150 nm nanowire/Ti/Au contact circuit (red) and the NiFe (7.5 μm wide)/Graphene/150 nm nanowire/Ti/Au contact circuit (blue) at 10 K. ( b ) Temperature dependence of zero-bias resistance for the NiFe/graphene contact (weakly insulating) and Au/Ti contact (metallic). Full size image 3T Hanle measurements The spin-injecting properties and spin-RA products of the NiFe/graphene tunnel barrier contacts were initially assessed using the 3T geometry in which a single FM contact is used to both generate and detect spin accumulation in the area of the NW immediately beneath the contact [24] , [25] , [31] . Here a current is applied to contacts 1 and 3 (see Fig. 3a ), and a voltage is measured across contacts 3 and 4. The injection of spin-polarized electrons from FM contact 3 produces a net spin accumulation in the Si nanowire described by the splitting of the spin-dependent electrochemical potential ( μ ), Δ μ = μ up − μ down , where μ up and μ down are the chemical potentials for the up- and down-spin electrons as shown in Fig. 3b . This spin splitting is detected as a voltage Δ V 3T = γ Δ μ /2 e , where γ ∼ 0.4 is the tunnelling spin polarization of the magnetic tunnel contact. When a magnetic field B z is applied along the surface normal and perpendicular to the electron spin direction, spin precession at the Larmor frequency ω L =gμ B B z /ħ results in a reduction of the net spin accumulation due to precessional dephasing (Hanle effect, Fig. 3b ) [42] . Here g is the Lande g -factor ( g =2 for Si), μ B the Bohr magneton and ħ is the reduced Planck’s constant. 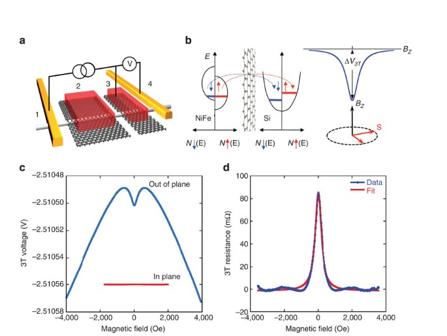Figure 3: 3T Hanle measurements. (a) Schematic of the 3T measurement; (b) simplified diagram illustrating spin injection from the NiFe across the graphene tunnel barrier producing spin accumulation in the Si NW and the Hanle spin precession measurement. N↑(E) and N↓ (E) are the majority and minority spin density of states, respectively. (c) Raw data for the normal (blue trace, magnetic field out of plane) and inverted (red trace, magnetic field in plane) 3T Hanle measurements for a 150-nm diameter NW at 10 K and −200 μA bias current (spin injection). (d) Same normal Hanle curve ascafter a quadratic background subtraction and plotted as resistance. The red line is a fit of the data. The voltage Δ V 3T ( B z ) decreases with B z with a Lorentzian lineshape given by [42] : Figure 3: 3T Hanle measurements. ( a ) Schematic of the 3T measurement; ( b ) simplified diagram illustrating spin injection from the NiFe across the graphene tunnel barrier producing spin accumulation in the Si NW and the Hanle spin precession measurement. N↑( E ) and N↓ ( E ) are the majority and minority spin density of states, respectively. ( c ) Raw data for the normal (blue trace, magnetic field out of plane) and inverted (red trace, magnetic field in plane) 3T Hanle measurements for a 150-nm diameter NW at 10 K and −200 μA bias current (spin injection). ( d ) Same normal Hanle curve as c after a quadratic background subtraction and plotted as resistance. The red line is a fit of the data. Full size image Fits to the data provide a lower bound for the effective spin lifetime τ s , which reflects the environment sampled by the spin directly beneath the FM tunnel barrier contact (note that this is not a measure of the intrinsic spin lifetime of Si [24] ). The raw data for the 3T Hanle measurements with the magnetic field applied out of plane (normal Hanle effect, blue trace) and in plane (inverted Hanle effect, red trace) are shown in Fig. 3c at 10 K for a bias current of −200 μA for which spin-polarized electrons are injected from the magnetic contact into the Si (spin injection condition). The normal Hanle signal appears as the dip near zero field superposed on a B 2 background. After subtracting this quadratic background, the data exhibit the expected Lorentzian lineshape as shown in Fig. 3d . Fits to the data using equation (1) yield a spin lifetime of 260±10 ps, a factor of 2 longer than that obtained in planar Si devices of similar doping level with either oxide [24] or graphene tunnel barrier contacts [26] . The corresponding spin diffusion length is given by L SD =[ D τ s ] 0.5 ∼ 350 nm, where D =0.00047, m 2 s −1 is the diffusion constant determined from fits to the NLSV Hanle data described below. No evidence for a Hanle-like signal is observed when the magnetic field is applied in-plane along the long axis of the magnetic contact. The appearance of such an ‘inverted’ Hanle effect has been attributed to precessional dephasing produced by random fringe fields arising from surface/interface roughness of the magnetic contact [43] , although other factors may contribute [44] . The absence of an inverted Hanle signal implies that the NiFe/graphene tunnel barrier produces a more uniform magnetic film and interface, which suppress such effects relative to that provided by the NiFe/oxide interface. Samples with non-magnetic reference contacts exhibit only a background signal. In a true one-dimensional (1D) structure, the spin lifetime should be significantly enhanced due to the discontinuous density of states that reduces available spin relaxation channels [45] . We indeed see a factor of 2 enhancement relative to bulk control samples. However, Si nanowires are expected to exhibit true 1D behaviour only for diameters < ∼ 10 nm (refs 46 , 47 ). The diameter of the nanowires used here and in measurements by other groups [32] , [33] , [34] , [35] , [36] are all much larger due to limitations in fabrication, and therefore too wide to exhibit an ideal 1D density of states and the corresponding full enhancement in spin lifetime. The fact that the Hanle-derived spin lifetime is not reduced relative to values obtained from similar measurements on bulk planar samples [24] , [26] indicates that surface scattering due to the much larger surface-to-volume ratio for the NW does not play a more significant role at these relatively high doping levels, or that another relaxation mechanism dominates. The Hanle-derived effective spin lifetime we measure is an order of magnitude shorter than the 2.5-ns lifetime obtained from electron spin resonance measurements on bulk samples of similar carrier density [48] . We attribute this to the proximity of the FM contact interface where magnetic fringe fields due to contact edges or closure domains may lead to strong local spin precession and dephasing [49] , [50] . In addition, spins can scatter at the FM contact interface, or readily diffuse between the Si and FM metal contact through the relatively transparent tunnel barrier. Enhancement of the spin lifetime previously seen in InGaAs nanowires was explained by a suppression of D’yakonov-Perel spin dephasing in semiconductors without crystalline inversion symmetry [51] . However, this mechanism is not applicable to Si due to the inversion symmetry of the diamond lattice. The amplitude of the measured spin resistance area product obtained from the 3T Hanle signal is significantly smaller than that predicted by the theory of spin injection into a semiconductor channel in the diffusive regime. The measured value is given by Δ V 3T (0) A / I b =2.6 mΩ μm 2 , where A and I b are the contact area and bias current, respectively. The contact area is taken to be the product of the contact width (200 nm) and the NW diameter (150 nm), although it may be geometrically much smaller than that due to the NW curvature. The amplitude predicted by the model of Fert and Jaffres for direct tunnelling [16] is given by γ 2 r 1 = γ 2 ( ρ L SD )=5.6 Ωμm 2 , where γ ∼ 0.4 is the tunnelling spin polarization of the magnetic tunnel contact, ρ =0.01 Ωcm is the NW resistivity and L SD ∼ 350 nm. The large discrepancy may be attributed to leakage currents, an overestimate of the actual tunnel contact area due to inhomogeneous tunnelling or an overestimate of the tunnelling spin polarization. Previous work has suggested that spin signals much larger than those predicted by theory may be due to spurious effects such as spin accumulation in localized interface states rather than in the semiconductor channel itself [52] , anomalous scaling [53] or magnetic field-modulated resonant tunnelling [54] . The fact that our experimental value is smaller than that predicted provides some evidence that such effects do not play a significant role in our devices. NLSV measurements We use the same samples in the NLSV geometry of Fig. 1a to demonstrate the generation and detection of pure spin current in the NW channel produced by the NiFe/graphene contacts. In these measurements, contacts 3 and 4 are biased such that spin-polarized electrons are injected from the narrow 200-nm contact 3 into the nanowire, producing a spin accumulation in the nanowire beneath the contact. Spin diffusion causes a pure spin current to flow in the nanowire towards contact 2, and a corresponding spin splitting of the electrochemical potential, Δ μ = μ up − μ down , can be detected as a voltage on contact 2. Note that the non-local detector contact 2 is unbiased and outside of the charge current path. This spin splitting Δ μ decreases exponentially with distance from the injecting contact 3 with a characteristic spin diffusion length L SD . The results are shown in Fig. 4a . The non-local resistance is defined to be the voltage measured at the non-local detector contact 2 divided by the bias current applied between contacts 3 and 4. An in-plane magnetic field is used to switch the magnetizations of the two electrodes independently due to their different coercive fields, producing parallel and antiparallel alignments. When the magnetizations of detector contact 2 and injector contact 3 are parallel, a low non-local resistance is measured, and when the magnetizations are antiparallel a high non-local resistance is measured—this is the classic signature of a NLSV device. 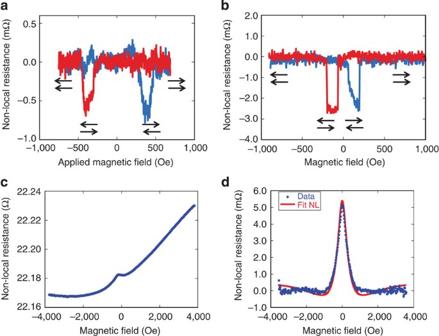Figure 4: NLSV and Hanle measurements. (a) NLSV data on 150 nm wide nanowire, contacts are 200 nm and 1 μm wide with a 200 nm edge-to-edge spacing. The arrows indicate the relative orientation of the magnetizations of the injector and detector contacts, and the blue and red traces indicate increasing and decreasing magnetic field sweeps. (b) NLSV on bulk Si sample with the same contact layout. (c) Raw NLSV Hanle data for the Si NW for parallel alignment of contacts 2 and 3. (d) Same NLSV Hanle data after background subtraction. All data are for a bias current of −200 μA atT=10 K, peak is 5 mΩ. A net change in the non-local resistance of ∼ 0.7 mΩ was measured at 10 K. Figure 4: NLSV and Hanle measurements. ( a ) NLSV data on 150 nm wide nanowire, contacts are 200 nm and 1 μm wide with a 200 nm edge-to-edge spacing. The arrows indicate the relative orientation of the magnetizations of the injector and detector contacts, and the blue and red traces indicate increasing and decreasing magnetic field sweeps. ( b ) NLSV on bulk Si sample with the same contact layout. ( c ) Raw NLSV Hanle data for the Si NW for parallel alignment of contacts 2 and 3. ( d ) Same NLSV Hanle data after background subtraction. All data are for a bias current of −200 μA at T =10 K, peak is 5 mΩ. Full size image The magnetizations of the two contacts reverse cleanly at well-defined coercive fields consistent with shape anisotropy, so that both parallel and antiparallel alignment of the injector/detector magnetizations are realized. We attribute this to the smooth bridging of the NW by the graphene layer as discussed above ( Fig. 1b–d ), producing a more gradual variation in the contact topography to which the NiFe film conforms. In contrast, magnetic metal/oxide tunnel contacts applied directly to the NW exhibit poorly defined switching characteristics attributed to local domain patterns arising from the more complex morphology created as the contact attempts to conform to the NW sidewalls [33] . The switching characteristics observed in Fig. 4a are comparable to those exhibited by planar NLSV devices with NiFe/graphene tunnel barrier contacts on bulk Si wafers [26] . Data for the planar Si NLSV samples are shown for comparison in Fig. 4b for a similar contact layout on a bulk Si wafer with a carrier concentration of 1 × 10 19 cm −3 . Application of an out-of-plane magnetic field causes the spins to precess and dephase as they diffuse towards the detector contact 2, and the non-local voltage decreases with increasing magnetic field due to this Hanle effect. The NLSV Hanle data are shown in Fig. 4c (raw) and Fig. 4d (after background subtraction), and can be modelled using the integral spin diffusion approach described in the literature [30] , [55] . The model fits the experimental data well, as shown by the red curve in Fig. 4d , and yields values for the diffusion constant D =0.00047, m 2 s −1 and the NLSV spin lifetime of 190±10 ps. This effective spin lifetime is shorter than the value of 260±10 ps obtained in the 3T geometry, although the reasons are unclear at present. Both values are shorter than the 10 ns reported at 8 K for NLSV structures grown by molecular beam epitaxy on silicon-on-insulator substrates exhibiting a 2 × 1/1 × 2 reflection high energy electron diffraction pattern [22] . This is consistent with the general expectation that air-exposed interfaces are likely to incorporate impurities resulting in spin scattering. The spin diffusion length is calculated as L SD =[ D τ s ] 0.5 ∼ 300 nm, which is significantly shorter than results reported previously [32] , [33] . However, these were based only on the amplitude of the NLSV data rather than direct determination of the spin lifetime provided by the Hanle measurements. The amplitude of the non-local Hanle signal measured at contact 2 is 1 μV or 5 mΩ, approximately an order of magnitude larger than expected based on the NLSV signal of 0.7 mΩ of Fig. 4a . In theory, it should be one-half of the NLSV amplitude. We do not understand this at present, but speculate that it may arise from some small leakage of the effective 3T signal originating at injector contact 3. The facts that the spin lifetimes (190 ps versus 260 ps) and the backgrounds observed in the raw data for the NLSV versus 3T Hanle measurements are very different indicates that the NLSV Hanle data are not dominated by potential leakage from the 3T signal. The geometrical enhancement predicted by the Jaffres and Fert model for very narrow spin channels occurs only when L SD is much larger than the width (or diameter), w , of the spin transport channel ( L SD >> w ) [56] , [57] , which is not the case for our devices ( L SD ∼ 300 nm, NW diameter w ∼ 100 nm). Also, as discussed above, we do not expect a significantly enhanced spin voltage arising from a lengthening of the spin lifetime unless the nanowire is a true 1D structure with a discrete density of states. This requires either long electron mean free paths or very narrow diameters (<10 nm for Si) [46] , [47] . Select samples with large 3T Hanle signals Some processing runs produced NW devices that yielded only 3T signals and no NLSV data, despite the fact that NW growth and device fabrication were done in nominally identical fashions (although months apart). Data were obtained on devices with a 7.5-μm wide single FM contact. For these devices, the Hanle signal was quite large and persisted to room temperature. 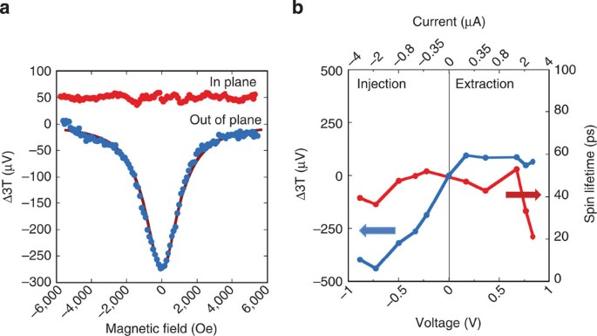Figure 5: Anomalously large signals from selected devices. (a) Normal (blue points) and inverted (red points) 3T Hanle data obtained atT=10 K and a bias current of −0.5 μA from a 150-nm diameter Si nanowire with a 7.5-μm wide contact. The solid red line is a fit to the normal 3T Hanle data, and yields a spin lifetimeτs=50 ps. A parabolic background has been subtracted. (b) Amplitude of the normal 3T Hanle signal (blue) and corresponding spin lifetime (red) as a function of bias. Figure 5a shows the normal (blue trace) and inverted (red trace) 3T Hanle voltage for a bias of −0.5 μA at 10 K (spin injection). A normal Hanle signal is clearly visible as a dip at zero field after a parabolic background has been subtracted. No evidence of an inverted Hanle signal is observed, providing further evidence that the graphene layer has a smoothing effect that reduces interface roughness of the NiFe injector and thus minimizes accompanying fringe fields. Control samples using non-magnetic contacts show small positive magnetoresistance consistent with a Lorentzian type of magnetoresistance, ruling out weak localization, which might be more prevalent for these lower dimensional samples [58] , [59] . Both the amplitude (550 Ω) and linewidth are much larger than those of corresponding data obtained from NW samples which showed NLSV signals ( Figs 3d and 4d ). Fits to this lineshape using equation (1) give a lower bound for τ s and yield a spin lifetime of ∼ 50 ps, much shorter than the 190–260 ps measured for NWs which also showed NLSV behaviour, and also shorter than previously reported on planar bulk silicon devices with similar carrier concentration (100–125 ps). Figure 5: Anomalously large signals from selected devices. ( a ) Normal (blue points) and inverted (red points) 3T Hanle data obtained at T =10 K and a bias current of −0.5 μA from a 150-nm diameter Si nanowire with a 7.5-μm wide contact. The solid red line is a fit to the normal 3T Hanle data, and yields a spin lifetime τ s =50 ps. A parabolic background has been subtracted. ( b ) Amplitude of the normal 3T Hanle signal (blue) and corresponding spin lifetime (red) as a function of bias. Full size image To better understand these data, we note that Aoki et al. [44] reported both normal/inverted 3T Hanle and NLSV measurements on n -type (5 × 10 19 cm −3 ) 80-nm thick Si films. At T =8 K, they observed a very broad normal 3T Hanle curve with a very narrow feature near zero field with an ∼ 100-Oe linewidth superposed on it. The broad component corresponded to a 42-ps spin lifetime, which was much shorter than the value they obtained from their NLSV Hanle measurements, similar to the situation we report here. They further showed that the magnitudes of both the broad normal 3T Hanle component and of the inverted 3T Hanle do not depend on the bias current, which is inconsistent with standard models of spin injection and accumulation, and suggests an alternate origin. All of their data were obtained for biases corresponding to spin extraction. There are several notable differences between their results and those we report. First, we see no inverted Hanle signal ( Fig. 5a ). Second, we observe no narrow feature near zero field in the normal 3T Hanle measurement, only the broad component shown in Fig. 5a . Third, we examine bias conditions corresponding to both spin injection and extraction. As shown in Fig. 5b , the amplitude of the normal 3T Hanle signal shows a pronounced dependence on bias for the full range examined for spin injection, consistent with theoretical expectations for spin injection/accumulation. However, it exhibits a rapid saturation for the conditions of spin extraction considered by Aoki et al. even though the I–V curve we measure shows no such saturation ( Fig. 2a ). This may be attributed in part to the bias dependence of the detection efficiency [60] , or to less efficient spin filtering due to reduced spin polarization of the NiFe density of states above the Fermi level [61] , [62] , or to the decrease we observe in the spin lifetime at the higher biases considered in Fig. 5b . Spin signals could be measured at room temperature, and a large spin resistance of 229 Ω still exists at 300 K. These values are two orders of magnitude larger than expected from the model of Fert and Jaffres. As noted earlier, previous work has suggested that anomalously large 3T spin signals may result from spin accumulation in localized interface states rather than in the semiconductor channel itself [52] , anomalous scaling [53] or magnetic field-modulated resonant tunnelling [54] . Further work is necessary to elucidate the origin of these large signals. In summary, we have utilized FM metal/graphene tunnel barriers to electrically inject and detect spin currents in silicon nanowire transport channels. The single-layer graphene provides a high-quality tunnel barrier with a low-resistance area product free of pinholes that smoothly bridges the nanowire. This results in clean magnetic switching characteristics for the magnetic contacts, and enables the first observation of Hanle spin precession of both spin accumulation in the nanowire in the 3T geometry, and of the pure spin current generated in the nanowire transport channel using the NLSV geometry. The Hanle data provide direct measurements of the spin lifetime and spin diffusion lengths in these nanoscale spintronic devices. By fitting the Hanle data, we obtain spin lifetimes of 260 ps with 3T measurements and 190 ps in the NLSV devices at 10 K, corresponding to spin diffusion lengths of 300–350 nm. As noted previously, Si nanowires are expected to exhibit true 1D behaviour only for diameters < ∼ 10 nm. The term nanowire typically refers to the geometry, not the electronic structure. The vast majority of investigations including the work reported here are on nanowires with diameters larger than 10 nm (refs 32 , 33 , 34 , 35 , 36 ), and these larger diameter nanowires are most relevant for the majority of applications. Achieving good contacts remains one of the largest technological barriers to exploiting geometrical nanowires, and in the 10–200-nm regime there are strong size-dependent effects arising from electrostatics [63] . Hence, the present study explores a highly relevant diameter regime, and the approach described is readily applicable to nanowires with diameters of 10 nm and below. Utilizing intrinsic 2D layers such as graphene or hexagonal boron nitride as tunnel contacts on nanowires offers many advantages over conventional materials deposited by vapour deposition (for example, Al 2 O 3 or MgO), enabling a path to highly scaled electronic and spintronic devices. Nanowire fabrication Si nanowires (NWs) were grown on SiO 2 layers seeded with Au nanoclusters. The reactor was evacuated to <100 mTorr, heated to ∼ 440 °C under Ar flow, and then Si NWs were grown for 5–10 min with a 10–80 s.c.c.m. flow of SiH 4 (10% in He), resulting in nanowires with a <111> growth axis [38] . The low density of defects is confirmed by high-resolution transmission electron microscopy. The wires were phosphorous doped to an electron concentration n ∼ 3 × 10 19 cm −3 . They were removed from the growth substrate by sonication and dispersed onto a Si 3 N 4 /Si substrate. Graphene growth and transfer Graphene was synthesized via low-pressure chemical vapour deposition on a copper foil substrate using methane gas [39] . The typical grain size of the graphene films is several hundred microns. The graphene/Cu samples were coated in PMMA and the Cu was etched in an ammonium persulfate-based solution. The remaining graphene/PMMA films were transferred into a deionized water bath before drying onto HF-etched Si nanowires and removing the PMMA with acetone. The quality of the graphene was assessed using Raman spectroscopy. The absence of the ‘D’ line ( ∼ 1,350 cm −1 ) associated with defects, and the widths and ratios of the ‘G’ ( ∼ 1,580 cm −1 ) and ‘2D’ ( ∼ 2,700 cm −1 ) lines confirm that the graphene is of high quality with minimal defects. Electrical measurements Electrical measurements were performed in a cryogen-free cryostat and electromagnet system. The integrity of the graphene tunnel barrier was confirmed by using typical I–V analysis procedures [41] , including successful fits of the I–V curves with the Brinkman–Dynes–Rowell model, and demonstrating a weak temperature dependence of the zero-bias resistance. The Hanle measurements were performed using an out-of-plane magnetic field either in 3T mode where one contact serves as both injector and detector, as depicted in Fig. 3a , or in a four-terminal NLSV configuration where contact 3 is the injector and contact 2 is the detector. The out-of-plane magnetic field produces precessional dephasing of the spin system in the Si NW, and at sufficiently high field suppresses any spin accumulation from the injector contact. The spin voltage measured at the detector is proportional to the spin polarization in the channel. The magnetic field dependence of this voltage is used as an indicator for the spin properties of the nanowire—the contact voltage decreases with increasing magnetic field, producing a pseudo-Lorentzian lineshape, and fits to this lineshape provide a measure of the spin lifetime. The non-local spin-valve measurement uses the four-terminal configuration. Here an in-plane magnetic field is used to switch the magnetization of contacts 2 and 3 independently. When the two contacts are aligned antiparallel, a low non-local voltage is measured, and when the two contacts are parallel aligned a high voltage is measured. How to cite this article: van ’t Erve, O. M. J. et al. Spin transport and Hanle effect in silicon nanowires using graphene tunnel barriers. Nat. Commun. 6:7541 doi: 10.1038/ncomms8541 (2015).